Arylcarboxylation of unactivated alkenes with CO2via visible-light photoredox catalysis Photocatalytic carboxylation of alkenes with CO 2 is a promising and sustainable strategy to synthesize high value-added carboxylic acids. However, it is challenging and rarely investigated for unactivated alkenes due to their low reactivities. Herein, we report a visible-light photoredox-catalyzed arylcarboxylation of unactivated alkenes with CO 2 , delivering a variety of tetrahydronaphthalen-1-ylacetic acids, indan-1-ylacetic acids, indolin-3-ylacetic acids, chroman-4-ylacetic acids and thiochroman-4-ylacetic acids in moderate-to-good yields. This reaction features high chemo- and regio-selectivities, mild reaction conditions (1 atm, room temperature), broad substrate scope, good functional group compatibility, easy scalability and facile derivatization of products. Mechanistic studies indicate that in situ generation of carbon dioxide radical anion and following radical addition to unactivated alkenes might be involved in the process. Carbon dioxide (CO 2 ), which is inexpensive, non-toxic, and recyclable, has been regarded as an ideal one-carbon feedstock to engage in chemical transformations for the synthesis of high value-added chemicals [1] , [2] , [3] , [4] . As carboxylic acids are a privileged functional group in biochemistry and polymer chemistry, it is highly important to develop direct and flexible methods for carboxylation with CO 2 [5] , [6] , [7] , [8] , [9] . In recent years, visible-light photocatalytic carboxylation with CO 2 has attracted much attention as an efficient, versatile, and sustainable strategy [10] , [11] , [12] , [13] , [14] , [15] . As alkenes are common functional group in organic compounds and bulk chemicals in industry, visible-light photocatalytic carboxylation of alkenes with CO 2 is of particular interest [16] , [17] , [18] , [19] , [20] , [21] , [22] , [23] , [24] , [25] , [26] , [27] , [28] , [29] . Notably, visible-light photoredox-catalyzed difunctionalizing carboxylation of alkenes with CO 2 has recently emerged as an important access to valuable carboxylic acids with diverse functionality and high step economy [22] , [23] , [24] , [25] , [26] , [27] , [28] , [29] . Many groups, including Martin, Wu, Li, Xi, and our group, have reported visible-light photoredox-catalyzed 1,2-difunctionalizing carboxylation of alkenes with CO 2 under mild conditions in high chemo- and regio-selectivities (Fig. 1a ) [22] , [23] , [24] , [25] , [26] , [27] , [28] , [29] . However, these methods are mainly limited to activated alkenes, such as styrenes and acrylates. The photocatalytic 1,2-difunctionalizing carboxylation of unactivated alkenes with CO 2 has not been disclosed yet. Fig. 1: Visible-light photocatalytic 1,2-difunctionalizing carboxylation of alkenes with CO 2 . a Visible-light photocatalytic 1,2-difunctionalizing carboxylation of activated alkenes with CO 2 . b Visible-light photocatalytic arylcarboxylation of unactivated alkenes with CO 2 . PC photocatalyst, EWGs electron-withdrawing groups. Full size image As well known, unactivated alkenes are more abundant and easily available in nature and industry than activated alkenes. However, it is challenging for unactivated alkenes to undergo photocatalytic carboxylations with CO 2 [30] , [31] , [32] , [33] , arising from high reductive potentials of both starting materials [34] , [35] , [36] , [37] , [38] , [39] and sluggish radical addition onto unactivated alkenes to generate alkyl carbon radicals [40] , [41] , [42] , [43] , [44] , [45] , [46] , [47] , [48] , [49] , which are less stable than those from activated alkenes. Inspired by our recent work on hydrocarboxylation of unactivated alkenes with CO 2 [33] , we further challenged us whether we could tune the chemoselectivity from C−H to C−C bonds formation based on similar carbon radical intermediates (Fig. 1b ). We hypothesized the in situ generation of CO 2 radical anion (CO 2 •− ) and following radical addition to unactivated alkenes would result in unstabilized alkyl carbon radicals, which could be further trapped by arenes to generate the C−C bonds. Final rearomatization could give the desired arylcarboxylation products. If successful, it will realize 1,2-difunctionalizing carboxylation of unactivated alkenes with CO 2 . Moreover, as it is redox-neutral and atom-economic based on the C−H functionalization, it will also provide a practical and sustainable strategy to access a wide range of polycyclic carboxylic acids, which are highly important but not easy to obtain via other methods (Fig. 2 ). Nevertheless, many challenges remain. For example, it is challenging for conversion of CO 2 into CO 2 •− due to the high reduction potential of CO 2 [E 1/2 (CO 2 /CO 2 •− ) = −2.21 V vs SCE] [50] . Moreover, the addition of nucleophilic CO 2 •− to electron-rich unactivated alkenes is a polarity-mismatched process [51] . In addition, hydrocarboxylation, arylthiolation, and other competitive side reactions would also hamper the desired difunctionalizing carboxylation. Fig. 2: Selected biologically active carboxylic acids and derivatives bearing polycyclic structures. Examples of biologically active compounds possessing polycyclic acids and derivatives motifs. Full size image Herein, we report our success in realizing the visible-light photoredox-catalyzed arylcarboxylation of unactivated alkenes with CO 2 (Fig. 1b ). A variety of tetrahydronaphthalen-1-ylacetic acids, indan-1-ylacetic acids, indolin-3-ylacetic acids, chroman-4-ylacetic acids and thiochroman-4-ylacetic acids are generated in high selectivities and moderate-to-good yields. Screening of reaction conditions As carboxylic acids with polycyclic structures are widely found in natural products, drugs and bioactive compounds (Fig. 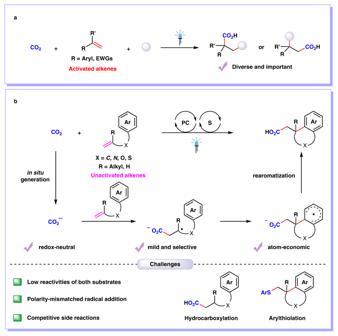Fig. 1: Visible-light photocatalytic 1,2-difunctionalizing carboxylation of alkenes with CO2. aVisible-light photocatalytic 1,2-difunctionalizing carboxylation of activated alkenes with CO2.bVisible-light photocatalytic arylcarboxylation of unactivated alkenes with CO2. PC photocatalyst, EWGs electron-withdrawing groups. 2 ) [52] , [53] , [54] , [55] , [56] , we initiated our project with 1a as standard substrate to generate tetrahydronaphthalen-1-ylacetic acid 2a as the desired product (Table 1 ). In the presence of fac -Ir(ppy) 3 ( Ir-1 ) as photocatalyst, 4- tert -butylthiophenol ( T1 ) as hydrogen atom transfer (HAT) catalyst and Cs 2 CO 3 as base (Please see the Supplementary Tables 1 – 5 in Supplementary Information ( SI) for more details), the desired arylcarboxylation product 2a was obtained in 66% yield with high selectivity (Entry 1). Control experiments revealed that photocatalyst, thiol catalyst, Cs 2 CO 3 , visible light, and CO 2 all played essential roles in the reaction (Entries 2–6). The use of p - t BuC 6 H 4 SK ( T2 ) instead of p - t BuC 6 H 4 SH ( T1 ) provided 2a in comparable yield (Entry 7). To our delight, PhMe 2 SiH turned to be a good additive that enhanced the yield of 2a to 86%, probably owing to the promotion of the CO 2 •− generation in the reaction (Entry 8) [57] . A variety of reaction conditions with other photocatalysts, solvents, HAT catalysts, bases, and silanes were also tested to give lower conversions and yields (Entries 9–14). Table. 1 Optimization of reaction conditions a Full size table Substrate scope Having established the optimized reaction conditions, we investigated the substrate scope (Fig. 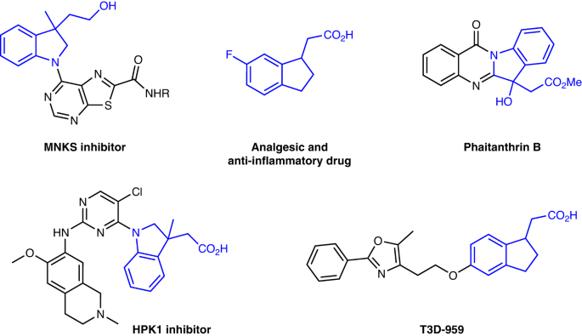Fig. 2: Selected biologically active carboxylic acids and derivatives bearing polycyclic structures. Examples of biologically active compounds possessing polycyclic acids and derivatives motifs. 3 ). A wide variety of electron-donating groups (EDGs) and EWGs were tolerant at the para -positions of the arene moiety, providing the desired products 2a – 2n in moderate-to-good yields. Substrates containing various functional groups, such as trifluoromethoxyl group ( 2d ), fluoro ( 2g ), amines ( 2i – 2k ), thioether ( 2l ) and amide ( 2m ), were smoothly converted to the corresponding products, thus allowing for downstream transformations. The efficiency of this protocol was not hampered by the ortho substituents on the phenyl ring, giving the corresponding arylcarboxylation products 2o – 2p in moderate-to-good yields. Substrates with different substituents on the aliphatic chain were also suitable for such a transformation, furnishing products 2q – 2t in 53–81% yields. When no ester group was present in the substrate, the carboxylative cyclization product 2u could also be obtained. To our delight, substrate 1v with tert -butyl group at the meta -position of the phenyl ring was tested in this reaction to give product 2v in 73% yield and sole regioselectivity owing to the steric hindrance effect. The substrate 1w bearing di-methoxyl groups also underwent the reaction smoothly to afford the arylcarboxylation product 2w in 77% yield. We were delighted to find that 5-exo cyclization process could also occur under such conditions, giving the indan-1-ylacetic acids 2x – 2z in moderate-to-good yields. We next turned our attention to 1,1-disubstituted unactivated alkenes as CO 2 coupling partners, which have rarely been used for photocatalytic cyclization reactions [58] . To our delight, this system also accomplished the 6-exo cyclizations to furnish carbocycles 2aa - 2ad containing the quaternary carbon centers in 48–63% yields. Fig. 3: Arylcarboxylation of unactivated alkenes with CO 2 to construct tetrahydronaphthalen-1-ylacetic acid and indan-1-ylacetic acid derivatives. a Standard reaction conditions (Table 1 , Entry 8) with yields of isolated carboxylic acids or methyl esters. b Esterification by MeI (0.4 mmol, 2.0 equiv. ), 65 °C, 3 h. Full size image As indoline derivatives are privileged structural motifs found in alkaloids [59] and clinical drugs [60] , seeking an efficient and simple approach for the construction of indolines is of continuous interest. Encouraged by the above results, we further turned our attention to selective carboxylation of N -protected allylanilines 3 with CO 2 to afford indolin-3-ylacetic acid derivatives 4 (Fig. 4 ). Mono-substituents on the aromatic ring had a negligible impact on these reactions, as the corresponding indoline derivatives 4a – 4g were obtained in satisfactory yields. Further investigations of the substrate scope showed that di- or tri-substituted N -protected allylanilines also delivered the corresponding indolin-3-ylacetic acid derivatives 4 h and 4i in synthetically useful yields. Fig. 4: Arylcarboxylation of unactivated alkenes with CO 2 to construct indolin-3-ylacetic acid derivatives. a Standard reaction conditions (Table 1 , Entry 8) with yields of isolated methyl esters. Full size image Inspired by above results, we wondered whether other kinds of valuable polycyclic carboxylic acids could be formed using this strategy. As chromanes and thiochromanes are widely distributed in nature and display a broad range of biological and pharmaceutical activities [61] , [62] , [63] , we further tested phenol- and thiophenol-derived alkenes 5 under standard reaction conditions. Fortunately, these substrates were also reactive to furnish the desired chroman-4-ylacetic acid and thiochroman-4-ylacetic acid derivatives 6a – 6d in 21–65% yields (Fig. 5 ). Fig. 5: Arylcarboxylation of unactivated alkenes with CO 2 to construct chroman-4-ylacetic acid and thiochromane-4-ylacetic acid derivatives. a Standard reaction conditions (Table 1 , Entry 8) with yields of isolated methyl esters. Full size image Synthetic applications In order to demonstrate the utility of this method, a gram-scale reaction and product derivatizations were performed (Fig. 6 ). The product 2a was obtained in 84% yield and gram scale, demonstrating the facile scalability of this reaction (Fig. 6a ). Then, we carried out the derivatization of 2a to illustrate potential synthetic applications (Fig. 6b ). Selective reduction of product 2a by using NaBH 4 produced the alcohol 7 in 92% yield [64] . Condensation between 2a and methyl glycinate hydro-chloride gave cyclic amide 8 in an excellent yield [65] . A practical decarboxylation of primary carboxylic acid 2a via synergistic photoredox and HAT catalysis was achieved in excellent yield [66] . And 2a could also participate in decarboxylative trifluoromethylation to give compound 10 in moderate yield [67] . Notably, compound 2a was easily transformed to the redox-active ester 11 [68] , which underwent C−P and C−S bonds formation through decarboxylative phosphination [69] and arylthiolation [70] , respectively. Fig. 6: Synthetic applications. a Gram-scale reaction. b Product derivatizations. Please see SI for experimental details. Gly-OMe·HCl glycine methyl ester hydrochloride. HOBt 1-hydroxybenzotriazole, EDCI 1-ethyl-3-(3-dimethylaminopropyl)carbodiimide, NPhth phthalimidyl, BTMG 2- tert -butyl-1,1,3,3-tetramethylguanidine, DMAP 4-dimethylaminopyridine. DCC Dicyclohexylcarbodiimide, PMDTA Pentamethyldiethylenetriamine. Full size image Mechanistic investigations To gain more insight into this reaction, a series of control experiments were conducted (Fig. 7 ). When the reaction was performed in the presence of various radical scavengers, such as 2,2,6,6-tetramethyl-1-piperidiny-1-oxy (TEMPO) or diphenyldiselenide (PhSeSePh), the formation of product 2a was completely inhibited with almost full recovery of 1a , indicating that radical process might be involved (Fig. 7a ). As the formation of reduction product 1a’ was not observed under nitrogen atmosphere, we believed that unactivated alkenes could not be reduced in the reaction (Fig. 7b ). The results of detecting of formate (HCO 2 − ) in the presence or absence of unactivated alkenes indicated that CO 2 •− could be generated from single electron reduction of CO 2 in the reaction (Fig. 7c ). Moreover, Stern-Volmer fluorescence quenching experiments showed that the excited state of the photocatalyst was quenched by the thiolate rather than unactivated alkenes (Fig. 7d ). Fig. 7: Mechanistic investigations. 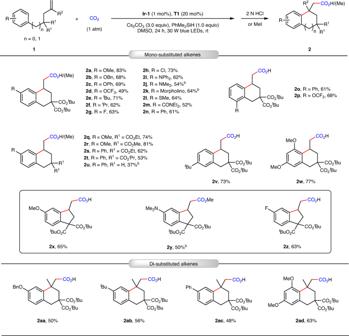Fig. 3: Arylcarboxylation of unactivated alkenes with CO2to construct tetrahydronaphthalen-1-ylacetic acid and indan-1-ylacetic acid derivatives. aStandard reaction conditions (Table1, Entry 8) with yields of isolated carboxylic acids or methyl esters.bEsterification by MeI (0.4 mmol, 2.0 equiv.), 65 °C, 3 h. a Radical trapping experiments. b Reduction of unactivated alkene 1a . c Detection of formate. d Stern-Volmer fluorescence quenching experiments. Full size image Based on the control experiments and previous studies [71] , [72] , [73] , a possible mechanism for the overall transformation of 1a is proposed (Fig. 8 ). The irradiation of photocatalyst fac -Ir III (ppy) 3 generates excited fac -*Ir III (ppy) 3 (E 1/2 *III/II = +0.31 V vs SCE), which can be reductively quenched by a catalytic thiolate to furnish fac -Ir II (ppy) 3 and a thiyl radical. Then, the Ir II species (E 1/2 III/II = −2.19 V vs SCE) [72] may engage in reducing CO 2 [E 1/2 (CO 2 /CO 2 •− ) = −2.21 V vs SCE] [50] via SET event to deliver CO 2 •− along with regeneration of fac -Ir III (ppy) 3 to close the photoredox catalytic cycle. The in situ generated CO 2 •− then undergoes radical addition to the C = C double bond of unactivated alkene of 1a to form an alkyl carbon radical A [30] , [33] , which is supposed to be quickly captured via cyclization to form the radical intermediate B . Finally, the carboxylate could be obtained via a HAT process of radical intermediate B with the thiyl radical, along with regeneration of the thiol catalyst [74] . The protonation during workup would afford the final product 2a . Meanwhile, the intermediate B might also undergo intermolecular HAT to deliver anti-Markovnikov hydrocarboxylation byproduct C [33] . In addition, we reason that the silane can serve as an additive to promote the generation of CO 2 •− from an alternative pathway (Please see Supplementary Fig. 18 in SI ) [57] . 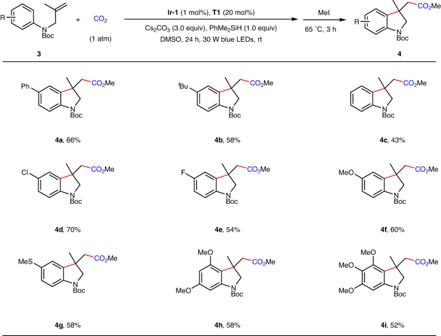Fig. 4: Arylcarboxylation of unactivated alkenes with CO2to construct indolin-3-ylacetic acid derivatives. aStandard reaction conditions (Table1, Entry 8) with yields of isolated methyl esters. At this stage, we could not exclude other alternative pathways (Please see SI for details) [75] , [76] . Fig. 8: Proposed mechanism. Proposed catalytic cycle for this synergistic catalyzed arylcarboxylation of unactivated alkenes with CO 2 . Full size image In summary, we have developed the visible-light photoredox-catalyzed arylcarboxylation of unactivated alkenes with CO 2 . This protocol provides an efficient and facile approach to an array of high-valued polycyclic carboxylic acids, such as tetrahydronaphthalen-1-ylacetic acids, indan-1-ylacetic acids, indolin-3-ylacetic acids, chroman-4-ylacetic acids and thiochroman-4-ylacetic acids. This reaction features mild reaction conditions, broad substrate scope, and good functional group compatibility. Moreover, the derivatization of products could afford diverse valuable polycyclic compounds, which are difficult to access via other protocols. Further applications of CO 2 •− and difunctionalizing carboxylation of unactivated alkenes are undergoing in our group. Synthesis of 2a-2z To an oven-dried Schlenk tube (25 mL) equipped with a magnetic stir bar was added the unactivated alkenes (0.2 mmol, 1.0 equiv. for solid substrates) and fac -Ir(ppy) 3 (1 mol%). The tube was moved into the glovebox where was added the Cs 2 CO 3 (0.6 mmol, 195.5 mg, 3.0 equiv.). The tube was sealed and removed from the glovebox, then evacuated and back-filled with CO 2 atmosphere for three times. liquid alkenes were added under CO 2 atmosphere followed by anhydrous DMSO (2 mL), PhMe 2 SiH (0.2 mmol, 27.3 mg, 31 μL, 1.0 equiv. ), 4- tert -butylthiophenol (0.04 mol, 6.7 mg, 7.0 μL, 20 mol%), and the tube was sealed at atmospheric pressure of CO 2 (1 atm). The reaction was stirred and irradiated with a 30 W blue LED lamp (1 cm away, with a cooling fan to keep the reaction temperature at 25–30 °C and keeping the reaction region located in the center of LEDs lamp) for 24 h. Upon completion of the reaction, the reaction mixture was diluted with 3 mL ethyl ester (EA) and quenched by 3 mL 2 N HCl. After adding 10 mL of H 2 O, the mixture was extracted by EA for five times and the combined organic phases were concentrated in vacuo. The residue was purified by silica gel flash column chromatography (Petroleum/EA/AcOH 10/1/ ~ 5/1 ~ /5/10.2%) to give the pure desired product. Synthesis of 2aa-2ad To an oven-dried Schlenk tube (25 mL) equipped with a magnetic stir bar was added the unactivated alkenes (0.2 mmol, 1.0 equiv. for solid substrates) and fac -Ir(ppy) 3 (1 mol%). The tube was moved into the glovebox where was added the Cs 2 CO 3 (0.6 mmol, 195.5 mg, 3.0 equiv.). The tube was sealed and removed from the glovebox, then evacuated and back-filled with CO 2 atmosphere for three times. liquid alkenes were added under CO 2 atmosphere followed by anhydrous DMSO (2 mL), PhMe 2 SiH (0.2 mmol, 27.3 mg, 31 μL, 1.0 equiv. ), 4- tert -butylthiophenol (0.04 mol, 6.7 mg, 7.0 μL, 20 mol%), and the tube was sealed at atmospheric pressure of CO 2 (1 atm). 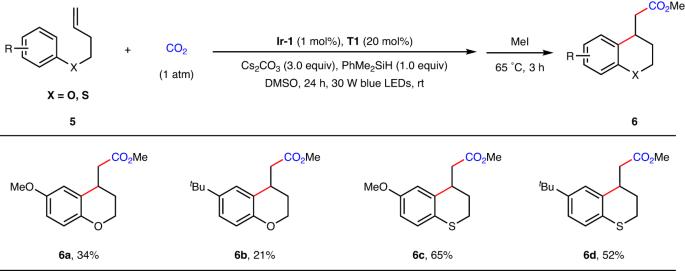Fig. 5: Arylcarboxylation of unactivated alkenes with CO2to construct chroman-4-ylacetic acid and thiochromane-4-ylacetic acid derivatives. aStandard reaction conditions (Table1, Entry 8) with yields of isolated methyl esters. The reaction was stirred and irradiated with a 30 W blue LED lamp (1 cm away, with a cooling fan to keep the reaction temperature at 25–30 °C and keeping the reaction region located in the center of LEDs lamp) for 24 h. Upon completion of the reaction, the reaction mixture was diluted with 3 mL EA and quenched by 3 mL 2 N HCl. After adding 10 mL of H 2 O, the mixture was extracted by EA for five times and the combined organic phases were concentrated in vacuo . The residue was purified by silica gel flash column chromatography (Petroleum/EA/AcOH 10/1/ ~ 5/1 ~ /5/10.2%) to give the pure desired product. Synthesis of 4a-4i To an oven-dried Schlenk tube (25 mL) equipped with a magnetic stir bar was added the unactivated alkenes (0.2 mmol, 1.0 equiv. for solid substrates) and fac -Ir(ppy) 3 (1 mol%). The tube was moved into the glovebox where was added the Cs 2 CO 3 (0.6 mmol, 195.5 mg, 3.0 equiv.). The tube was sealed and removed from the glovebox, then evacuated and back-filled with CO 2 atmosphere for three times. liquid alkenes were added under CO 2 atmosphere followed by anhydrous DMSO (2 mL), PhMe 2 SiH (0.2 mmol, 27.3 mg, 31 μL, 1.0 equiv. ), 4- tert -butylthiophenol (0.04 mol, 6.7 mg, 7.0 μL, 20 mol%), and the tube was sealed at atmospheric pressure of CO 2 (1 atm). The reaction was stirred and irradiated with a 30 W blue LED lamp (1 cm away, with a cooling fan to keep the reaction temperature at 25–30 °C and keeping the reaction region located in the center of LEDs lamp) for 24 h. Upon completion of the reaction, MeI (0.4 mmol, 25 μL, 2.0 equiv.) was added, the mixture was stirred at 65 o C for 3 h and then cooled to room temperature. The crude reaction mixture was diluted with 3 mL EA. After adding 10 mL of H 2 O, the mixture was extracted by EA for five times and the combined organic phases were concentrated in vacuo . The residue was purified by silica gel flash column chromatography (Petroleum/EA 60/1/ ~ 20/1) to give the pure desired product. Synthesis of 6a–6d To an oven-dried Schlenk tube (25 mL) equipped with a magnetic stir bar was added the unactivated alkenes (0.2 mmol, 1.0 equiv. for solid substrates) and fac -Ir(ppy) 3 (1 mol%). 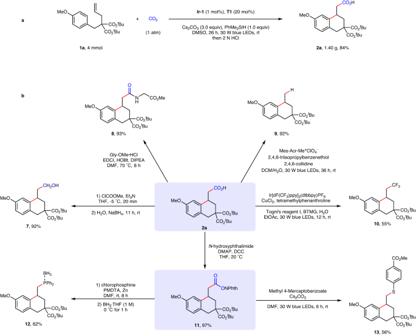Fig. 6: Synthetic applications. aGram-scale reaction.bProduct derivatizations. Please see SI for experimental details. Gly-OMe·HCl glycine methyl ester hydrochloride. HOBt 1-hydroxybenzotriazole, EDCI 1-ethyl-3-(3-dimethylaminopropyl)carbodiimide, NPhth phthalimidyl, BTMG 2-tert-butyl-1,1,3,3-tetramethylguanidine, DMAP 4-dimethylaminopyridine. DCC Dicyclohexylcarbodiimide, PMDTA Pentamethyldiethylenetriamine. The tube was moved into the glovebox where was added the Cs 2 CO 3 (0.6 mmol, 195.5 mg, 3.0 equiv.). The tube was sealed and removed from the glovebox, then evacuated and back-filled with CO 2 atmosphere for three times. liquid alkenes were added under CO 2 atmosphere followed by anhydrous DMSO (2 mL), PhMe 2 SiH (0.2 mmol, 27.3 mg, 31 μL, 1.0 equiv. ), 4- tert -butylthiophenol (0.04 mol, 6.7 mg, 7.0 μL, 20 mol%), and the tube was sealed at atmospheric pressure of CO 2 (1 atm). The reaction was stirred and irradiated with a 30 W blue LED lamp (1 cm away, with a cooling fan to keep the reaction temperature at 25–30 °C and keeping the reaction region located in the center of LEDs lamp) for 24 h. Upon completion of the reaction, MeI (0.4 mmol, 25 μL, 2.0 equiv.) was added, the mixture was stirred at 65 o C for 3 h and then cooled to room temperature. The crude reaction mixture was diluted with 3 mL EA. 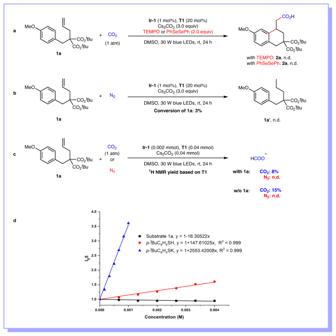Fig. 7: Mechanistic investigations. aRadical trapping experiments.bReduction of unactivated alkene1a.cDetection of formate.dStern-Volmer fluorescence quenching experiments. 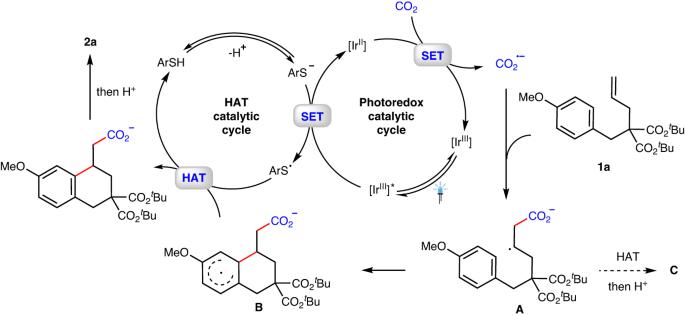Fig. 8: Proposed mechanism. Proposed catalytic cycle for this synergistic catalyzed arylcarboxylation of unactivated alkenes with CO2. After adding 10 mL of H 2 O, the mixture was extracted by EA for five times and the combined organic phases were concentrated in vacuo . The residue was first purified by silica gel flash column chromatography (Petroleum/EA 150/1/ ~ 60/1) to give the mixture and the yields were determined with CH 2 Br 2 as an internal standard. The desired arylcarboxylation products were further purified by preparative HPLC.